Antenna electrodes for controlling electroluminescence Optical antennas can control the emission from quantum emitters by modifying the local density of optical states via the Purcell effect. A variety of nanometallic antennas have been implemented to enhance and control key photoluminescence properties, such as the decay rate, directionality and polarization. However, their implementation in active devices has been hampered by the need to precisely place emitters near an antenna and to efficiently excite them electrically. Here we illustrate a design methodology for antenna electrodes that for the first time facilitates simultaneous operation as electrodes for current injection and as antennas capable of optically manipulating the electroluminescence. We show that by confining the electrically excited carriers to the vicinity of antenna electrodes and maximizing the optical coupling of the emission to a single, well-defined antenna mode, their electroluminescence can be effectively controlled. This work spurs the development of densely integrated, electrically driven light sources with tailored emission properties. Numerous studies on light-emitting diodes (LEDs) with large-area metallic electrodes showed that corrugating the electrode surface could enhance photon extraction from high refractive index emissive layers [1] , [2] , [3] , [4] , [5] , [6] , [7] , [8] , [9] , [10] . These improvements were attributed to the excitation of delocalized surface plasmon polaritons (SPPs) [11] or dielectric waveguide modes, and their subsequent scattering to free-space photon modes via the corrugations [12] . In the quest to realize increasingly compact and integrated electroluminescent (EL) devices, an opportunity to fashion the electrodes to support standing-wave SPP resonances emerged. The alternating currents associated with the oscillating SPPs enable effective radiation of the emitter's energy with tailored angular patterns and polarization properties through the use of the Purcell effect [13] , [14] , [15] . By optimizing both the optical process of local emission coupling to an antenna resonance and the electronic processes of charge injection and spatial carrier confinement, conventional large-area electrodes with undesirable mirror-like properties (when used as top contacts) can be redesigned to exhibit desirable emission features characteristic of optical antennas [15] , [16] , [17] , [18] , [19] , [20] , [21] , [22] . In this study, we start by reengineering conventional metallic stripe electrodes into optical antennas capable of controlling the EL from a quantum well (QW). In this effort, we leverage the significant knowledge base on the SPP modes supported by thin metal films and stripes. We then fabricate optimized antenna electrodes on planar QW and QW ridge devices emitting at 970 nm. We finish by experimentally demonstrating that antenna electrodes can indeed allow for effective control over the polarization and angular distribution of the QW emission in a fashion that agrees well with full-field simulations. Proposed plasmonic antenna-electrode platform The schematic of the antenna electrode is shown in Fig. 1a , which depicts two 20-nm-thick Au electrodes of different widths on a QW ridge. Each electrode supports a distinct SPP resonance when their widths are approximately an integer number, m , of half SPP wavelengths ( w ≈ m λ SPP /2) [23] , [24] , [25] as indicated by the magnetic field amplitude maps within the semiconductor. When current is injected into the QW via the antenna electrodes and the substrate, EL is emitted with an angular emission pattern that is characteristic to the electrode dimensions. We studied the EL properties of antenna electrodes placed on a flat QW and QW ridge based on In 0.16 Ga 0.84 As/GaAs with a peak emission wavelength around 970 nm at room temperature. Using standard processing techniques, we fabricated antenna electrodes (2 nm Ti/ 20 nm±2 nm Au) with widths of 60, 160 and 260 nm (±5 nm) on flat QW and electrodes with widths of 90, 190 and 290 nm (±5 nm) on top of 50-nm-high QW ridges (Methods). Each width corresponds to the first, second or third ( m =1, 2 or 3) resonance of the antenna. The bottom surface of the antenna electrode is spaced 10±3 nm above the QW for all samples. 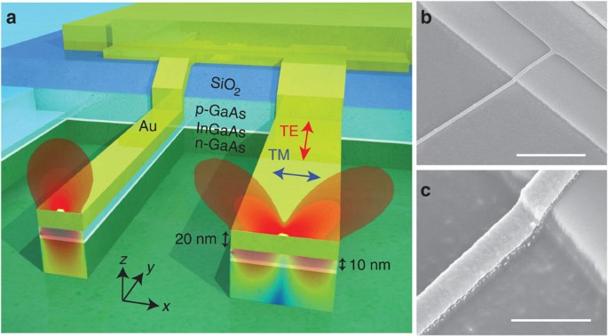Figure 1: Operation and implementation of the plasmonic antenna electrodes. (a) Schematic showing two antenna electrodes of different widths capable of injecting current into a QW ridge. The narrower electrode supports a half-wavelength SPP resonance (wλSPP/2) and the wider electrode supports a full-wavelength (wλSPP) resonance. The blue and red arrows indicate the direction of the electric field for the emission from modes that are transverse magnetic (TM) or transverse electric (TE). The magnetic field amplitudes for the supported TM modes are plotted underneath the antenna inside the QW ridge. The simulated angular light intensity distribution in the far-field is plotted above the antenna. (b) 45-degree-tilted scanning electron microscope (SEM) image of a fabricated device showing a narrow electrode connected to a large metal contact pad sitting on SiO2insulation. The white scale bar is 3 μm. (c) A high-magnification SEM image of the tip of the electrode taken at 10 keV. It shows the etched GaAs surface and the self-aligned antenna on top of the QW ridge. The white scale bar is 500 nm. Figure 1b,c show scanning electron microscope images of a fabricated antenna electrode on a QW ridge. All antenna electrodes are 35 μm in length to demonstrate uniformity in current spreading. Figure 1: Operation and implementation of the plasmonic antenna electrodes. ( a ) Schematic showing two antenna electrodes of different widths capable of injecting current into a QW ridge. The narrower electrode supports a half-wavelength SPP resonance ( w λ SPP /2) and the wider electrode supports a full-wavelength ( w λ SPP ) resonance. The blue and red arrows indicate the direction of the electric field for the emission from modes that are transverse magnetic (TM) or transverse electric (TE). The magnetic field amplitudes for the supported TM modes are plotted underneath the antenna inside the QW ridge. The simulated angular light intensity distribution in the far-field is plotted above the antenna. ( b ) 45-degree-tilted scanning electron microscope (SEM) image of a fabricated device showing a narrow electrode connected to a large metal contact pad sitting on SiO 2 insulation. The white scale bar is 3 μm. ( c ) A high-magnification SEM image of the tip of the electrode taken at 10 keV. It shows the etched GaAs surface and the self-aligned antenna on top of the QW ridge. The white scale bar is 500 nm. 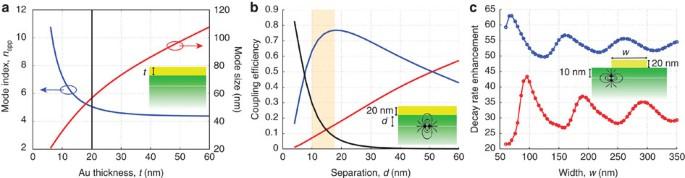Figure 2: Theoretical design guidelines for the antenna electrode operating at 970 nm wavelength. (a) Mode index and mode size as a function of metal thickness,t, for the asymmetric air-Au-GaAs SPP waveguide as shown schematically in the inset. The black line indicates the chosen metal thickness for all devices and subsequent calculations. (b) Coupling efficiency to continuum of propagating modes (red), SPP mode (blue) and lossy waves (black) for a randomly polarized dipole placed at varying distances,d, below the 20-nm-thick Au film, as depicted in the inset. The highlighted region indicates the location of the 8-nm-thick QW with respect to the bottom of the Au film. (c) Decay rate enhancement of a vertical dipole positioned 10 nm beneath the edge of the plasmonic stripe antenna, as shown in the inset, for the flat QW (blue) and QW ridge (red) calculated with 3D full-field simulations. Full size image Theoretical design guidelines for the antenna electrodes Figure 2 shows the analysis of the key optical design parameters including the antenna width ( w ), height ( t ) and thickness of the p-GaAs spacer layer ( d ) between the QW and electrode. The first two dictate the modal properties of the antenna and the third governs the coupling strength between the emitter and the antenna mode. To rapidly optimize these parameters, we treat the metal stripe as a truncated planar SPP waveguide for which the modal properties can be calculated analytically [26] . Figure 2: Theoretical design guidelines for the antenna electrode operating at 970 nm wavelength. ( a ) Mode index and mode size as a function of metal thickness, t , for the asymmetric air-Au-GaAs SPP waveguide as shown schematically in the inset. The black line indicates the chosen metal thickness for all devices and subsequent calculations. ( b ) Coupling efficiency to continuum of propagating modes (red), SPP mode (blue) and lossy waves (black) for a randomly polarized dipole placed at varying distances, d , below the 20-nm-thick Au film, as depicted in the inset. The highlighted region indicates the location of the 8-nm-thick QW with respect to the bottom of the Au film. ( c ) Decay rate enhancement of a vertical dipole positioned 10 nm beneath the edge of the plasmonic stripe antenna, as shown in the inset, for the flat QW (blue) and QW ridge (red) calculated with 3D full-field simulations. Full size image Figure 2a shows the calculated mode index ( n SPP ) and mode size for the air-Au-GaAs SPP waveguide (Methods). For Au thicknesses exceeding 30 nm, n SPP approaches the value for a single Au–GaAs interface SPP. Below 20 nm, n SPP rapidly increases as the SPPs on the two electrode surfaces (bottom and top) couple and produce a more confined mode with a reduced group velocity. As the emission enhancement is inversely proportional to the group velocity and the mode size from density of states considerations [27] , thin Au films are preferred from an optical perspective. However, from an electrical perspective, taking into account the sheet resistance, achievable film quality and increased electron scattering in nanoscale metal structures, we chose 20-nm-thick Au stripes for all devices (black line) to ensure uniform current spreading along the electrode. To optimize the spacer thickness, we calculated the coupling efficiency of a randomly polarized electrical dipole emitter to continuum of propagating radiation (free space and substrate emission), SPPs and high spatial frequency modes, known as lossy waves [26] (Methods) as a function of d ( Fig. 2b ). To maximize the coupling to SPPs and minimize the direct emission to the propagating continuum, we chose to space the 8-nm-thick QW 10 nm beneath the Au (highlighted region), just left of the point of maximum SPP coupling. This improves the far-field directivity at the cost of slightly more loss. To optimize the electrode width, we simulated the decay rate enhancement of a vertical dipole placed 10 nm underneath the antenna edge as a function of w in three-dimensional (3D) finite-difference time-domain (FDTD) simulations ( Fig. 2c ). The calculated enhancements oscillate with a periodicity corresponding to λ SPP /2 that is ~95 nm (consistent with n SPP ≈5 in Fig. 2a ) for both the antennas on the flat QW (blue) and on the QW ridge (red). There is a ~30 nm shift between peaks for the flat and ridge geometries, which can be attributed to a smaller SPP reflection phase at the terminations in the ridge structure. The maximum decay rate enhancement of ~63 may seem high for such a structure but is reasonable considering the calculation is performed for the optimal emitter positioning and polarization near the antenna. Although the partial removal of the high-index GaAs in the ridge structure results in lower overall enhancements (reduced number of modes in GaAs), the oscillation amplitude is ~50% larger compared with the flat geometry, indicating that a stronger transverse SPP resonance is excited across the width of the antenna ridge. This can be qualitatively understood by considering the larger index contrast between GaAs and the surrounding environment (air) for the ridge, which leads to higher reflectivity for SPPs. From 2D simulations of the same configurations for in-plane ( xz -plane) propagation, we indeed find larger enhancements for the ridge structure ( Supplementary Fig. S1 ). A beneficial consequence of the enhanced decay rate is a significantly faster modulation speed compared with conventional LEDs, which has been demonstrated elsewhere in both plasmonic [12] and photonic crystal systems [28] . In our presented devices, the spatial and polarization-averaged decay rate enhancements for the 90-nm-wide ridge antenna electrode is ~10 ( Supplementary Fig. S2 ), which would allow the QW LED to be electrically modulated at ~10 GHz (assuming an intrinsic lifetime of ~1 ns (ref. 29 )). Such fast modulation is desired for ultra-low power optical communication at high data rates. From the same 3D simulations, we also calculated the extraction efficiency (power radiated upwards from the top surface) for the ridge structure (~5.1%) and flat device (~3.5%). The rest of the EL power is either emitted into the substrate or guided down the length of the electrode as SPPs. This is significantly greater than the extraction efficiency of ~1.5% per air/GaAs output facet from a planar LED indicating that the electrodes are functioning as a radiating antenna instead of as a light-occluding mirror. Higher extraction efficiency can be readily achieved with 3D antenna array designs combined with thin-film flip-chip LED architectures. While a wide range of emission parameters such as temperature-dependent carrier lifetime, internal quantum efficiency and extraction efficiency are valuable performance measures directly related to our full-field simulations, optimization of these parameters to achieve the most efficient LED requires a holistic design of the epitaxial structure, electrode material, antenna periodicity, back reflector and encapsulation; this is not the objective of this report. Instead, we focus on the experimental demonstration of QW EL emission coupling to the antenna mode by imaging the polarization-dependent EL and angular radiation patterns from the antenna electrodes using an optical microscope to provide unequivocal signatures of tailored emission modification. 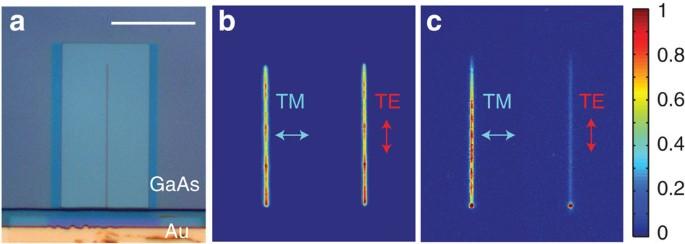Figure 3: Emission images from the antenna electrodes for different polarizations. (a) Optical bright field microscope image of a typical n-LED. The white scale bar is 20 μm. (b) TM and TE EL images of a 160-nm-wide antenna on the flat QW (no carrier confinement). (c) TM and TE EL images of a 190-nm-wide antenna on the QW ridge (with carrier confinement). The colour bar applies to the normalized EL intensities inbandcin linear scale. Antenna electrode-driven emission polarization behaviour Figure 3a is an optical image of a typical device. Figure 3b,c shows spatial EL maps that show uniform current spreading across the electrode. We measured the polarization ratio of the EL for 160-nm-wide flat devices ( Fig. 3b ) and 190-nm-wide ridge structures ( Fig. 3c ), both supporting the second-order resonance. It is clear that the emission from the flat QW device is unpolarized (TM/TE=1.0) while the QW ridge device radiates much more strongly in the TM polarization (TM/TE=16). The large polarization ratio for the ridge structure is indicative of efficient coupling to SPPs. To explain the result that the emission from the flat QW sample is unmodified, we consider the diffusion length of carriers in In 0.18 Ga 0.82 As QW to be l d ≈2.7 μm (ref. 29 ), which means the injected carriers can readily diffuse away from locations of enhanced local density of optical states (LDOS) near the antenna. For the ridge device, the finite width of the QW limits carrier diffusion and the radiative transitions are confined to directly underneath the antenna electrode, allowing strong SPP excitation. Figure 3: Emission images from the antenna electrodes for different polarizations. ( a ) Optical bright field microscope image of a typical n-LED. The white scale bar is 20 μm. ( b ) TM and TE EL images of a 160-nm-wide antenna on the flat QW (no carrier confinement). ( c ) TM and TE EL images of a 190-nm-wide antenna on the QW ridge (with carrier confinement). The colour bar applies to the normalized EL intensities in b and c in linear scale. Full size image Antenna electrode-driven emission radiation pattern The effects of carrier diffusion can also be observed by studying the radiation patterns of the ensemble emission; it causes optical transitions not only to occur directly underneath the antenna electrode where charges are injected, but also some distance away from the antenna. 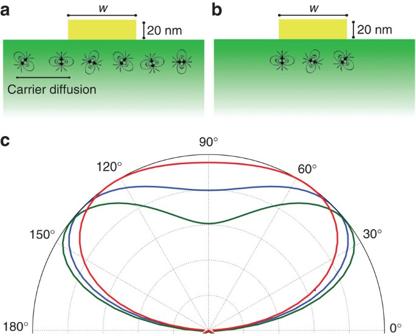Figure 4: Schematics and calculated TM angular radiation pattern illustrating the effects of increasing the carrier diffusion length. (a) With carrier diffusion, the emitters are located directly underneath the antenna as well as some distance away from the edge of the antenna. (b) Excited emitters are located only directly under the antenna to model the absence of carrier diffusion. (c) The radiation pattern for a 0-nm diffusion length (green) for an antenna electrode supporting the second-order resonance on flat QW shows two emission lobes at large angles. The patterns for 100 nm (blue) and 200 nm (red) lateral diffusion lengths exhibit increasingly less directive emission approaching that of the bare QW broadside emission. This is a significant effect even for the very short diffusion length of a few hundred nanometres (less than the diffraction limit of the microscope system). All three angular emission distribution curves are normalized to their maximum value. Figure 4a,b show schematics of situations with and without carrier diffusion. We chose to study an antenna electrode that supports the second-order resonance (160-nm-wide Au stripe) because its quadrupolar radiation pattern is significantly different from the Lambertian pattern of the bare QW. Figure 4c summarizes the simulated TM radiation patterns of an antenna excited by an ensemble of randomly polarized dipoles distributed only underneath the antenna (green), and with 100-nm (blue) or 200-nm diffusion lengths for the carriers (red). Without carrier diffusion, the emission pattern is clearly quadrupolar, evident from the two lobes at large angles away from the normal. Even with a minute diffusion length of 200 nm, the radiation pattern changes dramatically, exhibiting broadside dipolar emission, which is independent of the antenna design. Figure 4: Schematics and calculated TM angular radiation pattern illustrating the effects of increasing the carrier diffusion length. ( a ) With carrier diffusion, the emitters are located directly underneath the antenna as well as some distance away from the edge of the antenna. ( b ) Excited emitters are located only directly under the antenna to model the absence of carrier diffusion. ( c ) The radiation pattern for a 0-nm diffusion length (green) for an antenna electrode supporting the second-order resonance on flat QW shows two emission lobes at large angles. The patterns for 100 nm (blue) and 200 nm (red) lateral diffusion lengths exhibit increasingly less directive emission approaching that of the bare QW broadside emission. This is a significant effect even for the very short diffusion length of a few hundred nanometres (less than the diffraction limit of the microscope system). All three angular emission distribution curves are normalized to their maximum value. Full size image In our experiment, we compared the polarization-dependent radiation patterns from several different designs of antenna electrodes placed on the flat QW as well as the QW ridge to verify the effects of carrier diffusion and strong excitation of the antenna mode. The results are summarized in Fig. 5 . The upper and middle panels, respectively, show the experimentally measured and theoretically predicted patterns (970 nm wavelength) in the xz -plane (Methods). The TM polarization is plotted in blue and TE in red. The bottom panels show the corresponding simulated magnetic field amplitude around the antenna electrodes. The TE patterns are unchanged from that of the bare QW for all samples and serve as references. The patterns shown in Fig. 5a,b correspond to the same structures as Fig. 3b,c . Our simulations predict a two-lobed TM quadrupolar pattern for these antenna electrodes owing to the excitation of the full-wavelength SPP resonance. For the flat QW in Fig. 5a , the TM pattern resembles that of the bare QW, indicative of weak coupling to the SPP mode due to carrier diffusion away from the antenna. This observation is consistent with the unity polarization ratio in Fig. 3b . For the QW ridge in Fig. 5b , the TM pattern is strongly modified and the peak emission angle occurs at ~60° from the normal in agreement with calculations. However, the emission near the normal direction is not as strongly suppressed as predicted. This can be attributed to weaker SPP coupling owing to roughness scattering, finite EL bandwidth, higher loss in nanostructured metal [30] and absorption by the 2-nm Ti layer [31] . The black dashed line in Fig. 5b shows the theoretical TM pattern for an antenna with three times the tabulated metal loss [32] . With higher loss, the degree of EL suppression in the normal direction becomes weaker. To demonstrate the tunability in the angular pattern according to design, we show the experimental results for first-order (90 nm) and third-order (290 nm) antennas on the QW ridge in Fig. 5c,d . Both antennas exhibit emission patterns that are in excellent agreement with theory. The third-resonance antenna features a single lobe with enhanced directivity where the half-power beamwidth is ~70 degrees ( Supplementary Fig. S3 ). Such single-lobe emission [33] for higher-order resonance is characteristic of plasmonic antennas where λ SPP λ 0 . 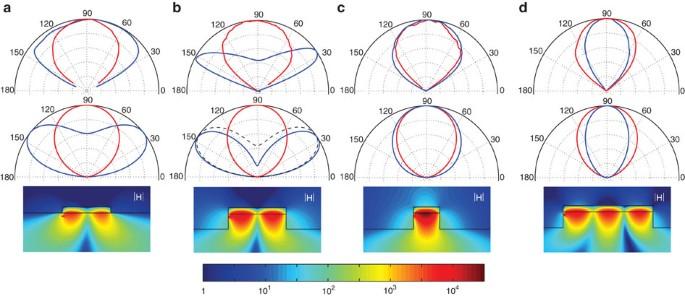Figure 5: Angular emission patterns for different antenna-electrode designs. Experimental (upper panels) and theoretical (middle panels) EL angular emission pattern for antennas of varying widths. TE polarization is shown in red and TM in blue. The corresponding simulated TM magnetic field amplitude for each antenna is displayed in the bottom panel on a log scale. (a) Second-order antenna on the flat QW. (b) Second-order antenna on the QW ridge. The black dashed curve shows the simulated TM pattern for an antenna with three times the tabulated metal loss data. (c) First-order antenna on the QW ridge. (d) Third-order antenna on the QW ridge. Figure 5: Angular emission patterns for different antenna-electrode designs. Experimental (upper panels) and theoretical (middle panels) EL angular emission pattern for antennas of varying widths. TE polarization is shown in red and TM in blue. The corresponding simulated TM magnetic field amplitude for each antenna is displayed in the bottom panel on a log scale. ( a ) Second-order antenna on the flat QW. ( b ) Second-order antenna on the QW ridge. The black dashed curve shows the simulated TM pattern for an antenna with three times the tabulated metal loss data. ( c ) First-order antenna on the QW ridge. ( d ) Third-order antenna on the QW ridge. Full size image With the use of antenna electrodes, a high degree of control over the EL properties of QW LEDs can be achieved. Their successful operation requires detailed optimization of electronic and optical processes, which hinges on the targeted generation and confinement of excitons near the antenna electrode and the careful design of the antenna geometries. This EL process is much more efficient compared with photoluminescence, which suffers greatly in carrier excitation efficiency owing to the size mismatch between the pump laser spot and the antenna. Moreover, rapid lateral carrier diffusion in the QW ( l d w ) upon electrical injection enables preferential recombination at locations near the electrode with the highest LDOS. This provides a practical advantage over QD or fluorescent molecule PL where carriers are spatially trapped, in which case the emitter must be precisely placed at the field intensity maximum. While metal losses associated with SPPs limit the efficiency of the LED, it is still possible to increase the efficiency of an LED provided that the radiative efficiency of the antenna is higher than the intrinsic quantum efficiency of the emitting material [21] . In this study, a very-high-efficiency InGaAs/GaAs QW is used; thus, the presence of the antenna would necessarily decrease the radiative quantum efficiency. However, efficiency improvements owing to the presence of plasmonic antennas can be expected in other commercial LED materials such as high Al content AlGaInP/GaAs QW emitting in the 590 nm regime where the internal quantum efficiency can be as low as ~13% (ref. 34 ). The demonstrated antenna electrodes facilitate excitation of strong SPP resonances, uniform current spreading and an ultra-compact device footprint. By leveraging the rapid development of new optical antenna designs, electrically driven and modulated optical sources with tailored emission properties may be realized. More generally, the presented antenna electrodes are part of a newly emerging class of structures capable of performing electronic and optical functions at the same time and in the same physical space. In devices that employ such structures, the traditional spatial boundary between electronic and photonic elements is disappearing and new opportunities for ultra-dense integration emerge. Calculations of the SPP mode and decay rate enhancement To obtain the mode index and mode size for the SPP mode, we numerically solve the dispersion relation of the asymmetric three-layer waveguide. The mode index is defined as n SPP =Re{ k SPP / k 0 }, where k SPP is the complex propagation constant of the SPP and k 0 is the free space propagation constant. The mode size is defined as t +0.5/γ GaAs +0.5/γ air where t is the Au film thickness and γ GaAs,air are the magnitudes of the field decay wavevectors into the GaAs and air. The theoretical decay rate enhancement of a dipole near a Au film of finite thickness is calculated using the forced damped harmonic oscillator model [26] . Contributions to the total decay rate enhancement owing to the excitation of continuum of propagating radiation, SPPs and lossy waves are obtained by first computing the decay rate enhancement as a function of the magnitude of the in-plane wavevector and identifying regions of small to large wavevectors (propagating continuum, SPP and lossy waves) with respect to k 0 ( Supplementary Figs S4 and S5 and Supplementary Methods ). Full-field electromagnetic simulations We performed full-field FDTD simulations [35] to model the resonance behaviour and radiation pattern of stripe antenna electrodes at a single free space wavelength of 970 nm. Although the LED has a ~50-nm emission bandwidth, we assume that all of it couples to a single broadband antenna mode ( Supplementary Fig. S6 ). The decay rate enhancement of dipoles near antenna electrodes of varying width is computed in 3D simulations, where we normalize the time-averaged total power flow emitted from the dipole near an antenna by the power output of the same current source placed in homogeneous GaAs. For each antenna resonance width, we calculate the angular emission pattern due to ensemble electric dipole excitation 10 nm beneath the antenna in 2D simulations. We ran a separate simulation for each dipole orientation ( x , y and z ) at each x -position in steps of 4 nm to mimic randomly polarized and positioned emitters. For each simulation, the near-field distribution around the antenna is converted to their equivalent surface currents, which are then used in a near-to-far-field transformation algorithm to produce the angular radiation pattern [36] . Substrate effects are accounted for using the transfer matrix method [37] . Radiated power as a function of angle from individual simulations is summed to obtain the ensemble emission pattern ( Supplementary Methods ). Owing to the symmetry of the stripe, the calculated angular pattern in 2D is equivalent to full 3D simulations for emission in the plane where the azimuthal angle is zero ( xz -plane, Supplementary Fig. S7 and Supplementary Discussion ). Sample fabrication The QW structure was grown by molecular beam epitaxy on an n-doped GaAs substrate and consists of a 500-nm n-doped Al 0.95 Ga 0. 05 As layer, a 50-nm n-doped GaAs layer, an 8-nm In 0.16 Ga 0.84 As QW surrounded by 20 nm GaAs barriers and a 30-nm p-doped GaAs layer. The doping densities for the n-GaAs and p-GaAs are 5×10 18 cm −3 and 1×10 19 cm −3 , respectively. A 200-nm SiO 2 layer is deposited on the wafer by plasma-enhanced chemical vapour deposition then wet etched with HF to transfer a photoresist pattern forming square insulation pads. Electron beam-evaporated 15 nm Cr/200 nm Au square contact pads are defined on the SiO 2 by photoresist lift-off. Selective area plasma etching (BCl 3 , Cl 2 ) of the wafer is used to expose n-GaAs substrate, onto which Au/Ge/Ni/Au is evaporated and annealed at 450 °C to form the n-contact. The top p-GaAs surface is plasma-etched to reduce the spacer layer to the desired thickness (~10 nm). The 2 nm Ti/20 nm Au antenna p-electrode is defined and connected to the large contact pad by electron beam lithography, 45-degree-tilted electron beam evaporation and lift-off. The sample is dipped in 20:1 buffered oxide etch to remove the native oxide on GaAs after electron beam lithography and before metal deposition. This concludes the fabrication of the flat QW samples. For the QW ridge samples, a final plasma-etching step is performed using the antenna electrode as a hard mask to remove the excess QW, thus forming a self-aligned electrode on the QW ridge. Experimental setup The fabricated antenna electrodes on QW LED are wirebonded ( Supplementary Fig. S8 ) and electrically driven with a pulsed voltage source. The circuit is terminated with a 50 Ω resistor. The 10 ns, 2 MHz voltage pulses are varied between 4–6 V ( Supplementary Fig. S9 ). The EL is imaged in a microscope setup with a polarizer using a X100, numerical aperture=0.9 objective (collection angle ~64 degrees) and detected with a Pixis 1024 thermoelectrically cooled Si CCD. The average current is measured concurrently using a Keithley picoammeter. For 35-μm long devices, the current typically range from a few hundred nA to 1 μA (current density of 10–20 A cm −2 , Supplementary Fig. S10 ). To measure the radiation pattern of the device, we defocus the microscope setup by 5 μm above the sample to image the lateral spread of the EL in real space. As there is a single emitting region in the xz -plane normal to the length of the electrode, we can convert the EL intensity in the x -direction to angular radiation pattern without the need for deconvolution. A cos( θ ) correction apodization factor is applied to ensure the differential area on the CCD plane and the polar arc stay equal as required by energy conservation for our imaging system, which satisfy the sine condition [38] ( Supplementary Figs S11 and S12 ). How to cite this article: Huang, K. C. Y. et al . Antenna electrodes for controlling electroluminescence. Nat. Commun. 3:1005 doi: 10.1038/ncomms1985 (2012).